Direct recognition of homology between double helices of DNA inNeurospora crassa Chromosomal regions of identical or nearly identical DNA sequence can preferentially associate with one another in the apparent absence of DNA breakage. Molecular mechanism(s) underlying such homology-dependent pairing phenomena remain(s) unknown. Using Neurospora crassa repeat-induced point mutation (RIP) as a model system, we show that a pair of DNA segments can be recognized as homologous, if they share triplets of base pairs arrayed with the matching periodicity of 11 or 12 base pairs. This pattern suggests direct interactions between slightly underwound co-aligned DNA duplexes engaging once per turn and over many consecutive turns. The process occurs in the absence of MEI3, the only RAD51/DMC1 protein in N. crassa , demonstrating independence from the canonical homology recognition pathway. A new perspective is thus provided for further analysis of the breakage-independent recognition of homology that underlies RIP and, potentially, other processes where sequence-specific pairing of intact chromosomes is involved. Chromosomal regions of identical or nearly identical DNA sequence can preferentially associate with one another in the apparent absence of DNA breakage and recombination. The genome-wide synapsis of homologous chromosomes in somatic nuclei of the fruit fly provides the archetype of such ‘break-independent pairing’ [1] . Additional examples include transient associations of homologous loci in mammalian somatic nuclei [2] , break-independent pairing of homologous chromosomes in meiosis [3] , [4] , [5] , [6] , [7] and repeat-directed DNA modifications in fungi [8] , [9] . The molecular mechanism(s) underlying these phenomena remain(s) an unsolved mystery of chromosome biology [10] . Break-independent pairing has been proposed to occur in vivo by direct DNA/DNA contacts [11] , [12] , RNA-mediated co-localization [13] or DNA-guided protein/protein interactions [14] . Different and/or multiple mechanisms might contribute in different systems. A mechanism involving direct DNA/DNA contacts is supported by in vitro studies [15] , [16] , [17] , [18] , [19] and by the existence of two related homology-sensing phenomena in filamentous fungi, RIP [8] (repeat-induced point mutation) and methylation-induced premeiotically [9] , wherein any duplication of ca. 0.4 kbp or longer undergoes cytosine methylation (methylation-induced premeiotically) or mutation (RIP) during a developmental stage that precedes the fusion of haploid nuclei at the onset of meiosis. A conserved group of putative cytosine methyltransferases responsible for the observed modifications has been identified [20] , [21] , but the actual homology sensing mechanism has remained elusive. In this study, we have explored the DNA sequence requirements for RIP in N. crassa by analysing distributions of mutations induced by strategically designed duplication constructs. Our RIP detection constructs all comprised a pair of DNA repeats separated by a short linker region. Each construct was integrated into a haploid strain A (Fungal Genetics Stock Center (FGSC) #9720 (refs 22 , 23 )) as a replacement of the wild-type allele of the cyclophilin gene csr-1 whose disruption confers selectable resistance to cyclosporin A [24] , [25] . RIP was triggered by mating primary homokaryotic transformants with a wild-type haploid strain B (FGSC #4200 (ref. 22 )) to produce a large number of haploid progeny spores. RIP mutations, specifically C-to-T (C/T) and G-to-A (G/A) transitions, were detected by sequencing the entire construct in a random sample of germinated cyclosporin-resistant repeat-carrying spores. Mutations were counted over the total sequenced region and, separately, over the longest invariant region shared by all constructs in a given experiment. Mutation counts from two or more crosses carrying the same repeat construct (replica crosses) were combined into a single empirical distribution. The equality of empirical distributions was evaluated by the two-sided Kolmogorov–Smirnov (K-S) test with the exact P -value calculated by permutation analysis. We show that RIP is triggered by short units of homology interspersed with a matching periodicity of 11 or 12 bp that slightly exceeds the 10.5-bp periodicity of relaxed B-DNA. The size of the minimal effective homology recognition unit is 3 bp. Participating DNA segments must be able to co-align along their lengths, and at least ∼ 150 bp of sequence identity are required to initiate mutation. In addition, RIP proceeds normally in the absence of MEI3, the only RAD51/DMC1 protein encoded in the N. crassa genome, demonstrating independence from the canonical homology recognition pathway. These and other results strongly suggest that intact double-stranded DNA molecules can engage in direct sequence-specific interactions in vivo , with a triplet of DNA base pairs as the likely fundamental recognition unit. RIP mutation strongly depends on homology length Our starting constructs contained direct repeats of 155–802 bp separated by a linker region of 0.7 kbp ( Fig. 1a,b ; Supplementary Figs 1 and 2 ). The 802-bp duplication induced a very strong RIP response, with 3041 C/T and 4067 G/A transitions (but no other types of mutations) identified in a sample of 24 sequenced spores. Gradually, restricting homology to 155 base pairs reduced mutation to a nearly undetectable level, where only 3 G/A transitions were found among 48 sequenced spores. This relationship was reflected in both the number of mutated DNA strands ( Fig. 1c ) and in the total number of mutations in the invariant region ( Fig. 1d ). Although the number of mutated strands may be related to the probability of forming an effective pairing interaction, the total number of mutations depends on this and other factors including the stability and dynamics of existing interactions as well as the number of mutable cytosines within a given repeat system. Despite these complexities, the number of mutations accurately reflected the extent of homology over the experimentally amenable range, thus encouraging its use for quantifying the RIP response. 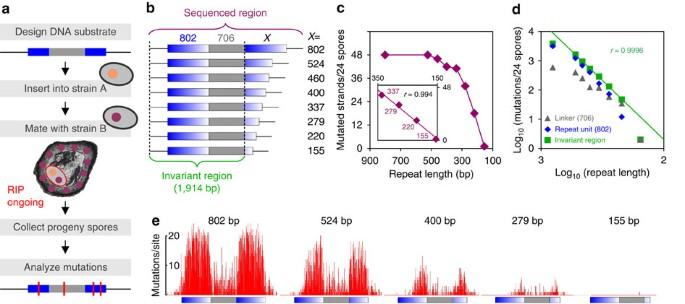Figure 1: Repeat-induced point mutation (RIP) strongly depends on homology length. (a) RIP is quantified by the number of mutations in a random sample of germinated spores. RIP substrates are introduced into haploid nuclei of Strain A (filled circles, orange). Maternal homokaryotic tissues originate from wild-type Strain B (filled circles, magenta). RIP occurs in heterokaryotic cells (outlined in red) containing nuclei of both parental strains. The heterokaryotic cell and the nuclei are not drawn to scale. (b) Direct perfect repeats of graded length assayed for RIP inc–e. The total sequenced region and the longest sub-region that is invariant among all constructs are indicated. (c) The total number of mutated DNA strands for repeat constructs inb. The number of spores analysed for each construct is provided inTable 1. (d) The total number of mutations in the invariant region (green) and its two non-overlapping segments: 802-bp (blue, some or all of which is part of the repeat unit) and the 706-bp (grey, linker). Regression analysis is based on mutation counts over the invariant region (1,914 bp) and includes the medium (524–220 bp) repeat range.rrepresents Pearson’s correlation coefficient. (e) Mutation profiles of selected repeat constructs. Figure 1: Repeat-induced point mutation (RIP) strongly depends on homology length. ( a ) RIP is quantified by the number of mutations in a random sample of germinated spores. RIP substrates are introduced into haploid nuclei of Strain A (filled circles, orange). Maternal homokaryotic tissues originate from wild-type Strain B (filled circles, magenta). RIP occurs in heterokaryotic cells (outlined in red) containing nuclei of both parental strains. The heterokaryotic cell and the nuclei are not drawn to scale. ( b ) Direct perfect repeats of graded length assayed for RIP in c – e . The total sequenced region and the longest sub-region that is invariant among all constructs are indicated. ( c ) The total number of mutated DNA strands for repeat constructs in b . The number of spores analysed for each construct is provided in Table 1 . ( d ) The total number of mutations in the invariant region (green) and its two non-overlapping segments: 802-bp (blue, some or all of which is part of the repeat unit) and the 706-bp (grey, linker). Regression analysis is based on mutation counts over the invariant region (1,914 bp) and includes the medium (524–220 bp) repeat range. r represents Pearson’s correlation coefficient. ( e ) Mutation profiles of selected repeat constructs. Full size image Intriguingly, as the extent of homology decreased from 802 to 155 bp, a greater proportion of mutations accumulated in the linker region, to the point when all mutations induced by the 155-bp duplication were located between the repeat units ( Fig. 1e ; Table 1 ). Although RIP had been shown to spread into adjacent single-copy sequences [26] , such strong mutation of the linker region was unexpected. Analysis of 150 spores containing the 220-bp duplication, the shortest repeat length for which statistically interpretable data could be obtained, showed that instances of strong, seemingly processive mutation occurred much more frequently than expected from a Poisson-like process ( Fig. 2a ). Yet, partitioning of individual mutations into repetitive and single-copy regions was independent of the total number of mutations found together on the same strand ( Fig. 2b ), suggesting that mutation of the linker reflected the intrinsic nature of the repeat recognition process. Table 1 Repeat constructs analysed in this study. 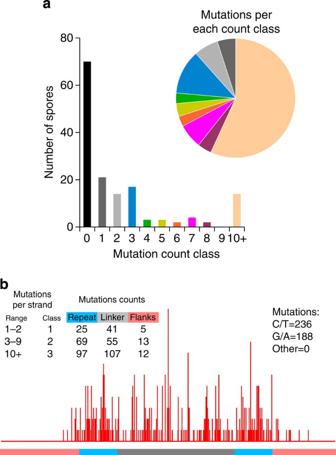Figure 2: Mutation of direct repeats containing 220 bp of perfect homology. (a) 424 mutations in 99 mutated strands were found among 150 sequenced spores. Spores were classified by the number of mutations over the total sequenced region. The number of spores (histogram) and the number of mutations (pie chart) per each class are shown. If the distribution of mutation counts followed a Poisson model (expected under the null assumption of independence of individual mutation events), the variance-to-mean ratio (VMR, distributed as the reduced chi-square under the Poisson model), would be equal to 1. VMR was found to be 30.98, significantly larger than 1 (P<1 × 10−6), indicating strong over-dispersion of mutation counts. (b) Mutation profile summarizes C/T and G/A mutations in 150 sequenced spores including the 24 spores analysed earlier (Fig. 1). To determine whether ample mutation of the linker region was associated with accidental bursts of repeat-induced point mutation (RIP) activity, every mutation was assigned two attributes: (i) its location in the construct, being either in the repeat unit, or the linker, or the flanking region, and (ii) the total number of mutations found together on the same stand. The data did not reveal any relationship between the number of mutations on a given strand and their partitioning into single-copy or repetitive regions (P=0.11, Fisher’s Exact test), suggesting that accidental bursts of RIP activity did not preferentially affect the linker region. Full size table Figure 2: Mutation of direct repeats containing 220 bp of perfect homology. ( a ) 424 mutations in 99 mutated strands were found among 150 sequenced spores. Spores were classified by the number of mutations over the total sequenced region. The number of spores (histogram) and the number of mutations (pie chart) per each class are shown. If the distribution of mutation counts followed a Poisson model (expected under the null assumption of independence of individual mutation events), the variance-to-mean ratio (VMR, distributed as the reduced chi-square under the Poisson model), would be equal to 1. VMR was found to be 30.98, significantly larger than 1 ( P <1 × 10 −6 ), indicating strong over-dispersion of mutation counts. ( b ) Mutation profile summarizes C/T and G/A mutations in 150 sequenced spores including the 24 spores analysed earlier ( Fig. 1 ). To determine whether ample mutation of the linker region was associated with accidental bursts of repeat-induced point mutation (RIP) activity, every mutation was assigned two attributes: (i) its location in the construct, being either in the repeat unit, or the linker, or the flanking region, and (ii) the total number of mutations found together on the same stand. The data did not reveal any relationship between the number of mutations on a given strand and their partitioning into single-copy or repetitive regions ( P =0.11, Fisher’s Exact test), suggesting that accidental bursts of RIP activity did not preferentially affect the linker region. Full size image Interrupted homology does not impede mutation We next asked if RIP was impeded by discontinuous homology. For this purpose, the original 220-bp construct was modified by including in each repeat unit an additional 200-bp segment, one copy of which remained invariant (‘Ref’), whereas the other (‘Test’) was altered as desired ( Fig. 3a ). Pairing of these partially homologous segments was expected to be initiated and/or stabilized within the adjacent 220-bp region of perfect homology, allowing detection of relatively subtle interactions. Mutation of the original 220-bp construct and the modified construct containing unrelated reference and test segments ( Fig. 3b , Test=green fluorescent protein) was statistically equivalent ( P =0.47, two-sided K-S test based on the total sequenced region, mutation counts for the 220-bp construct are based on the extended sample of 150 spores). Yet, a very strong RIP response was observed when the 200-bp segments were made identical ( Fig. 3b , Test=Ref). Introducing a region of heterology in the middle of the test segment, which was otherwise identical to the reference, had no effect on RIP ( Fig. 3c ), demonstrating its robust tolerance to some discontinuous homology. Because poly(dA:dT) tracts were shown to act as universal nucleosome repelling signals [27] , this result also suggested that homology recognition for RIP involved nucleosome-free segments of DNA. 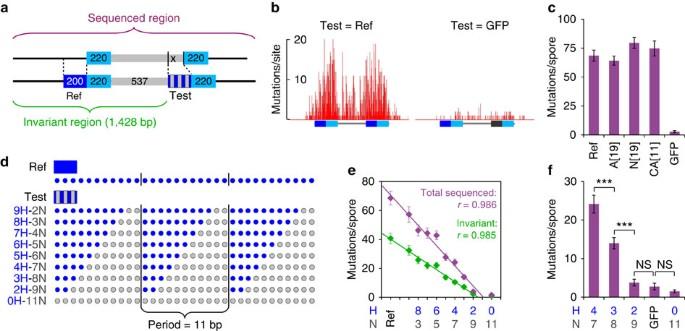Figure 3: Short periodic tracts of homology induce efficient repeat-induced point mutation. (a) The general structure of repeat constructs analysed inb–f. Each bipartite repeat unit contains 220 base pairs of perfect homology (turquoise) and 200 base pairs of interrupted homology (blue and blue/grey, corresponding to reference (Ref) and test segments, respectively). Only the test segment is allowed to vary between constructs. (b) Mutation profiles for situations of perfect homology (Test=Ref) and random homology (Test=green fluorescent protein (GFP)). Each mutation profile summarizes C/T and G/A transitions found over the entire sequenced region in 30 spores obtained from a single cross. (c) The number of mutations over the total sequenced region for repeat constructs carrying a region of heterology in the middle of the 200-bp test sequence that was otherwise identical to the reference. A[19], a 19-bp dA:dT tract; N[19], a 19-bp tract of random sequence; CA[11], CpA dinucleotide repeated 11 times. (d) Schematic representation of tested partial homologies with the matching periodicity of 11 bp: blue, matched bases, grey, random mismatched bases. (e) The number of mutations in the total sequenced (magenta) and the invariant (green) regions corresponding to test segments ind. Regression analysis excludes 0H-11N.rrepresents Pearson’s correlation coefficient. The number of analysed crosses and spores is provided inTable 1. (f) Statistical analysis of critical partial homologies. Mutation count distributions are compared by the two-sided Kolmogorov–Smirnov test: ***P<0.001; NS,P≥0.05. The number of analysed crosses and spores is provided inTable 1. Error bars represent s.e.m. Figure 3: Short periodic tracts of homology induce efficient repeat-induced point mutation. ( a ) The general structure of repeat constructs analysed in b – f . Each bipartite repeat unit contains 220 base pairs of perfect homology (turquoise) and 200 base pairs of interrupted homology (blue and blue/grey, corresponding to reference (Ref) and test segments, respectively). Only the test segment is allowed to vary between constructs. ( b ) Mutation profiles for situations of perfect homology (Test=Ref) and random homology (Test=green fluorescent protein (GFP)). Each mutation profile summarizes C/T and G/A transitions found over the entire sequenced region in 30 spores obtained from a single cross. ( c ) The number of mutations over the total sequenced region for repeat constructs carrying a region of heterology in the middle of the 200-bp test sequence that was otherwise identical to the reference. A[19], a 19-bp dA:dT tract; N[19], a 19-bp tract of random sequence; CA[11], CpA dinucleotide repeated 11 times. ( d ) Schematic representation of tested partial homologies with the matching periodicity of 11 bp: blue, matched bases, grey, random mismatched bases. ( e ) The number of mutations in the total sequenced (magenta) and the invariant (green) regions corresponding to test segments in d . Regression analysis excludes 0H-11N. r represents Pearson’s correlation coefficient. The number of analysed crosses and spores is provided in Table 1 . ( f ) Statistical analysis of critical partial homologies. Mutation count distributions are compared by the two-sided Kolmogorov–Smirnov test: *** P <0.001; NS, P ≥0.05. The number of analysed crosses and spores is provided in Table 1 . Error bars represent s.e.m. Full size image Short periodic tracts of homology induce efficient RIP Several models have been proposed in which homology sensing could occur between intact DNA duplexes [18] , [28] , [29] , and pairing of interspersed homologies has been demonstrated experimentally [18] . It thus seemed possible that homology recognition for RIP could involve short units of identical base pairs spaced intermittently with an appropriate periodicity. To evaluate this possibility, we designed test segments that matched the reference over short tracts of contiguous base pairs phased at 11-bp intervals approximating the 10.5 bp per turn of B-DNA ( Fig. 3d ). A strong linear relationship between the tract length and the number of mutations over the invariant and the total sequenced regions was observed ( Fig. 3e ). Only tracts of 3 bp or longer were capable of significantly increasing RIP mutation ( Fig. 3f ). We analogously examined test sequences containing 3-bp or 4-bp tracts phased at 11-bp intervals but beginning at a different position along the reference DNA (3H-8N′ and 4H-7N′, Fig. 4a ). These segments induced mutation as efficiently as the original ones ( Fig. 4b ), demonstrating the centrally important capacity of RIP to detect DNA homology per se rather than a particular combination of sequence motifs. Deleting every second homology unit in test segments 5H-6N and 7H-4N decreased mutation by the factor of four ( Fig. 4a,c ), indicating that the availability of pairing interactions at nearly every 11-bp unit was optimal for RIP. 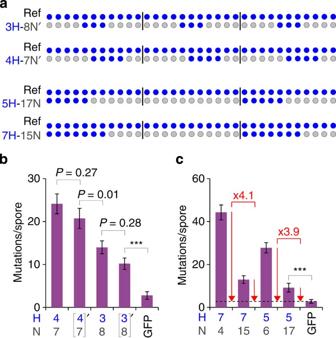Figure 4: Isolated periodic tracts of homology are recognized irrespectively of their nucleotide composition. (a) Schematic representation of tested partial homologies. 3H-8N′ shares 17% gross random homology with 3H-8N; 4H-7N′ shares 10.5% gross random homology with 4H-7N. (b) The number of mutations corresponding to segments containing 3-bp (3H-8N versus 3H-8N') and 4-bp (4H-7N versus 4H-7N′) tracts of homology arrayed with the 11-bp periodicity. (c) The number of mutations corresponding to test segments with every second homology unit removed. Data represent the mean number of mutations (per spore) over the total sequenced region. The number of analysed crosses and spores is provided inTable 1. Error bars represent s.e.m. Mutation count distributions are compared by the two-sided Kolmogorov–Smirnov test: ***P<0.001. GFP, green fluorescent protein. Figure 4: Isolated periodic tracts of homology are recognized irrespectively of their nucleotide composition. ( a ) Schematic representation of tested partial homologies. 3H-8N′ shares 17% gross random homology with 3H-8N; 4H-7N′ shares 10.5% gross random homology with 4H-7N. ( b ) The number of mutations corresponding to segments containing 3-bp (3H-8N versus 3H-8N') and 4-bp (4H-7N versus 4H-7N′) tracts of homology arrayed with the 11-bp periodicity. ( c ) The number of mutations corresponding to test segments with every second homology unit removed. Data represent the mean number of mutations (per spore) over the total sequenced region. The number of analysed crosses and spores is provided in Table 1 . Error bars represent s.e.m. Mutation count distributions are compared by the two-sided Kolmogorov–Smirnov test: *** P <0.001. GFP, green fluorescent protein. Full size image Homology units must be arrayed with matching periodicities If homology recognition for RIP involves juxtaposition of short tracts of identical sequence along intact DNA helices, then RIP should not be stimulated by tracts arrayed with periodicities deviating from ∼ 10.5 bp. Thus, we also examined pairs of 200-bp segments in which 3-bp units of homology occurred at periodicities of 10, 12 or 13 base pairs ( Fig. 5a ). While the 12-bp periodicity produced a strong increase in RIP mutation, comparable to the 11-bp periodicity, 10-bp and 13-bp periodicities did not yield a statistically significant signal ( Fig. 5b,c ). These results supported the notion that repeats interacted in a basic duplex state and also suggested that the involved duplexes could be slightly under-wound, thus favouring periodicities slightly longer than that of relaxed B-DNA. 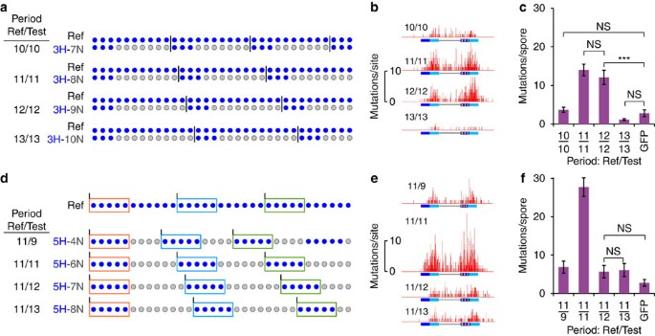Figure 5: Short periodic tracts of homology must be arrayed with the matching periodicity. (a) Ref/Test repeat pairs with 3-bp tracts of homology arrayed with matching periodicities of 10, 11, 12 and 13 bp. (b) Representative mutation profiles of repeat constructs ina. (c) The number of mutations for repeat constructs ina. (d) Repeat pairs with 5-bp tracts of homology arrayed with non-matching periodicities of 11 versus 9, 11 versus 12 and 11 versus 13 bp as compared with the original (matching) periodicity of 11 versus 11 bp. (e) Representative mutation profiles of repeat constructs ind. (f) The number of mutations for repeat constructs ind. Data represent the mean number of mutations (per spore) over the total sequenced region. The number of analysed crosses and spores is provided inTable 1. Error bars represent s.e.m. Mutation count distributions were compared by the two-sided Kolmogorov–Smirnov test: ***P<0.001; NS,P≥0.05. Each mutation profile summarizes all C/T an G/A mutations found over the entire sequenced region in 30 spores obtained from a single cross. GFP, green fluorescent protein. Figure 5: Short periodic tracts of homology must be arrayed with the matching periodicity. ( a ) Ref/Test repeat pairs with 3-bp tracts of homology arrayed with matching periodicities of 10, 11, 12 and 13 bp. ( b ) Representative mutation profiles of repeat constructs in a . ( c ) The number of mutations for repeat constructs in a . ( d ) Repeat pairs with 5-bp tracts of homology arrayed with non-matching periodicities of 11 versus 9, 11 versus 12 and 11 versus 13 bp as compared with the original (matching) periodicity of 11 versus 11 bp. ( e ) Representative mutation profiles of repeat constructs in d . ( f ) The number of mutations for repeat constructs in d . Data represent the mean number of mutations (per spore) over the total sequenced region. The number of analysed crosses and spores is provided in Table 1 . Error bars represent s.e.m. Mutation count distributions were compared by the two-sided Kolmogorov–Smirnov test: *** P <0.001; NS, P ≥0.05. Each mutation profile summarizes all C/T an G/A mutations found over the entire sequenced region in 30 spores obtained from a single cross. GFP, green fluorescent protein. Full size image This scenario further predicts that little or no increase in RIP mutation should occur if homologous tracts were placed with two different periodicities along the interacting molecules. To this end, we examined constructs containing a particular set of pentanucleotides with the 11-bp periodicity in the reference segment and the same set of pentanucleotides but arrayed with a periodicity of 9, 12 or 13 bp in the test segment ( Fig. 5d ). All combinations with non-matching periodicities (11/10, 11/12 and 11/13) were similarly ineffective in promoting RIP ( Fig. 5e,f ). It is particularly notable that the 11/12 combination did not increase RIP levels above background, despite the fact that 11/11 and 12/12 combinations were both highly effective ( Fig. 5c ). Thus, two DNA molecules that contain the same sequence of short matching tracts can be recognized as homologous, if and only if those tracts are arrayed with the optimal periodicity of 11 or 12 bp. The number of triplet frames predicts RIP mutation Appropriately spaced tracts of homology increase RIP mutation proportionally to their tract lengths ( Fig. 3e ). Although this relationship could reflect a trivial dependence on the total amount of homology, that possibility is not easily reconciled with the notion of a direct interaction between co-aligned DNA duplexes, which should be limited to only a few base pairs per turn. An alternative interpretation is that longer tracts provide more possible phases for alignment of elementary interaction units. The unit of three base pairs is the shortest tract of homology capable of increasing mutation above background ( Fig. 3f ). Correspondingly, if the elementary recognition unit were a triplet of base pairs, test segments 4H-7N and 6H-5N would have the potential to align with the reference segment by 2 and 4 alternative frames, respectively ( Fig. 6a , cases i and ii, in red). More generally, the number of triplet frames and the gross amount of homology are linearly proportional to the tract length for any test segment containing periodic uninterrupted units of homology ( Table 1 , in red). Thus, the observed linear dependence of RIP mutation on homology tract length could be explained by the number of potential frames as easily as by overall homology content. 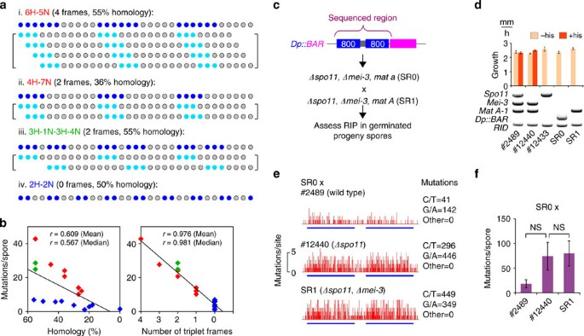Figure 6: Repeat-induced point mutation (RIP) is proportional to the number of triplet frames and does not require MEI3 (RAD51). (a) (i–iv) For each indicated Test segment (red, green or blue), all potential frames for aligning Test and Ref segments by triplets with the matching periodicity of 11 bp are given. The total number of such frames and overall homology between Test and Ref segments are indicated. Lines (i) and (ii) (red): two partial homologies analysed inFig. 3d,e. Line (iii) (green): a Test segment that contains as much overall homology as (i) and as many triplet frames as (ii). Line (iv) (blue): a Test segment that provides no triplet frames, but contains more overall homology than (ii) and nearly as much overall homology as (i) and (iii). (b) The mean number of mutations over the total sequenced region for constructs inTable 1(blue, red and green) plotted against the amount of overall homology (left panel) or the number of triplet frames as defined ina(right panel).rrepresents Pearson’s correlation coefficient. Correlation coefficients for the mean and the median values were computed separately. (c) Strategy for examining the role of MEI3 in RIP (Methods). Strains SR0 and SR1 were produced from a cross between strains #12433 (Δmei-3) and #12440 (Δspo11), which along with reference wild-type strain #2489 were obtained from the Fungal Genetics Stock Center22. (d) Strains used incwere phenotyped and genotyped by PCR. PCR bands correspond to wild-type alleles or theDp::BARduplication. TheΔmei-3genotype is verified by the histidine sensitivity assay. (e) Mutation profiles summarize 10 spores analysed from each cross. (f) The mean number of mutations (per spore) over the total sequenced region for the crosses shown ine. Mutation counts were compared by the two-sided Kolmogorov–Smirnov test: NS,P≥0.05. Error bars represent s.e.m. Figure 6: Repeat-induced point mutation (RIP) is proportional to the number of triplet frames and does not require MEI3 (RAD51). ( a ) (i–iv) For each indicated Test segment (red, green or blue), all potential frames for aligning Test and Ref segments by triplets with the matching periodicity of 11 bp are given. The total number of such frames and overall homology between Test and Ref segments are indicated. Lines (i) and (ii) (red): two partial homologies analysed in Fig. 3d,e . Line (iii) (green): a Test segment that contains as much overall homology as (i) and as many triplet frames as (ii). Line (iv) (blue): a Test segment that provides no triplet frames, but contains more overall homology than (ii) and nearly as much overall homology as (i) and (iii). ( b ) The mean number of mutations over the total sequenced region for constructs in Table 1 (blue, red and green) plotted against the amount of overall homology (left panel) or the number of triplet frames as defined in a (right panel). r represents Pearson’s correlation coefficient. Correlation coefficients for the mean and the median values were computed separately. ( c ) Strategy for examining the role of MEI3 in RIP (Methods). Strains SR0 and SR1 were produced from a cross between strains #12433 ( Δmei-3 ) and #12440 ( Δspo11 ), which along with reference wild-type strain #2489 were obtained from the Fungal Genetics Stock Center [22] . ( d ) Strains used in c were phenotyped and genotyped by PCR. PCR bands correspond to wild-type alleles or the Dp::BAR duplication. The Δmei-3 genotype is verified by the histidine sensitivity assay. ( e ) Mutation profiles summarize 10 spores analysed from each cross. ( f ) The mean number of mutations (per spore) over the total sequenced region for the crosses shown in e . Mutation counts were compared by the two-sided Kolmogorov–Smirnov test: NS, P ≥0.05. Error bars represent s.e.m. Full size image To distinguish between these two possibilities, we examined RIP in a situation where the number of triplet frames and the extent of homology were uncoupled. We designed a test sequence ‘3H-1N-3H-4N’ whose 11-bp periodic unit comprised two matching trinucleotides separated by a single mismatch, presenting gross homology of 55% in two triplet frames ( Fig. 6a : iii, green). 3H-1N-3H-4N promoted RIP mutation at the same level as canonical test sequences 4H-7N and 4H-7N′ that also contain two triplet frames but only 36% gross homology. Conversely, 3H-1N-3H-4N promoted RIP at approximately half the level of 6H-5N that presents the same amount of homology (55%) but twice as many triplet frames ( Table 1 ). Because the 1-bp separation between homology units might be insufficient to isolate them from each other, another test segment was designed to contain the 3-bp homologies separated by the 2-bp mismatch (‘3H-2N-3H-3N’). This test segment induced mutation analogously to 3H-1N-3H-4N ( P =0.51; Fig. 6b ; Table 1 , in green). As additional controls, we designed a test sequence ‘2H-2N’ containing 50% gross homology but no triplet frames ( Fig. 6a : iv, blue), and also re-examined cases in which matching by triplets was precluded ( Table 1 , blue). None of these test segments increased mutation nearly as strongly as 3H-8N', whose single frame yielded the lowest significant increase in RIP mutation recorded in this study ( Fig. 4b ). Overall, the number of triplet frames, rather than the overall level of homology, was the best predictor of RIP response ( Fig. 6b ), supporting the idea that the relevant variable was the number of unique phases available for aligning partially homologous DNA segments. RIP does not require MEI3 (RAD51) Triplet-based interactions are fundamental to the canonical homology recognition pathway mediated by the conserved RecA proteins RAD51 and DMC1 (ref. 30 ). Although RIP was shown to occur independently of one meiotic gene, mei-2 (refs 31 , 32 ), it remained unclear if RAD51 and DMC1 proteins were involved in RIP. We therefore examined the role of MEI3, the only RAD51/DMC1 protein encoded in the N. crassa genome [33] , [34] , in RIP using homozygous Δspo11, Δmei-3 crosses. Although the transesterase SPO11 is universally required for making recombination-initiating double-strand breaks in meiosis, a homozygous cross between Neurospora Δspo11 strains is still partially fertile [35] , and the Δspo11 mutation is expected to suppress the meiotic lethality of Δmei-3 . We generated Δspo11, Δmei-3 strains of opposite mating types and ectopically transformed the mat a strain with a 800-bp direct duplication of a metazoan gene AvHsp82 (ref. 36 ; Fig. 6c ). This approach allowed us to examine mutation of ‘naive’ DNA that had never encountered MEI3 protein. Crosses between the two Δspo11, Δmei-3 strains SR0 and SR1 ( Fig. 6c,d ) produced many viable spores containing the repeat cassette, as expected. Sequence analysis of these spores revealed strong RIP mutation ( Fig. 6e,f ). We conclude that MEI3 is not required for any aspect of RIP, including homology sensing. RIP depends on global disposition of interacting repeats The strong dependence of RIP on the length of homology ( Fig. 1c,d ) suggests that sequence information is sensed cumulatively over several hundred base pairs. If so, the overall repeat configuration should play a crucial role. We examined this possibility using a modified version of the basic 337-bp construct ( Fig. 1b ) in which the linker region was reduced from 706 to 303 bp to facilitate sequence analysis ( Fig. 7a , constructs i versus ii). This change slightly increased the level of RIP ( Fig. 7b , right, constructs i versus ii). In this modified context, RIP occurs at the same level regardless of whether the 337-bp repeats are present in direct or inverted orientation ( Fig. 7 , constructs ii versus iii). However, a dramatic dependence on overall repeat geometry emerges when the 337-bp repeats, present in inverted orientation, are flanked by 500-bp segments of partial homology (4H-7N). Although inverted partial homologies trigger very little RIP mutation by themselves ( Fig. 7 , construct iv), their mutation is strongly enhanced by the presence of perfect repeats in the same, inverted, orientation. Many mutations accumulate along the 4H-7N segments for up to 300–400 bp to either side of the perfect repeat. In striking contrast, when the flanking imperfect repeats are present in direct orientation on either side of the nucleating inverted repeat, where simple extension of the nucleation is impossible, mutations now occur essentially only within the region of perfect homology, at the same level seen in the absence of any flanking partial homology ( Fig. 7 , constructs v and vi). By implication, propagation of RIP from the nucleating interaction into the adjacent partially homologous regions requires continuous co-alignment of the participating segments. 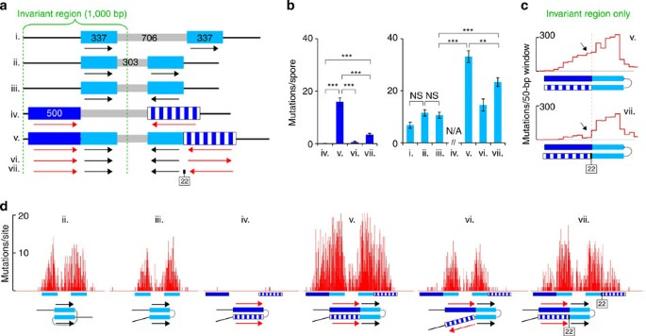Figure 7: Repeat-induced point mutation (RIP) depends on global disposition of interacting repeats. (a) Analysed constructs contain one or more of the following elements positioned, as shown, to either side of a 707-bp or a 303-bp linker region (grey): 337 bp of perfect homology (turquoise) in direct or inverted orientation; 500 bp of partial homology 4H-7N (blue and blue/white) in direct or inverted orientation, either alone or adjacent to 337 bp of perfect homology in inverted orientation, and with or without 22 bp of random sequence inserted between the perfect and partial homology segments. (b) The number of mutations within the partial homology repeat (left panel) and the perfect homology repeat (right panel) in the invariant region. For (ii-vii), corresponding mutation profiles shown ind. ***P<0.001; **P<0.01; NS,P≥0.05; ns,P-value fluctuates around 0.05. Error bars represent s.e.m. (c) Mutation density profiles for constructs (v) and (vii) reveal the effect of the 22-bp insertion at junction between perfect and imperfect inverted repeat units. The invariant region (1,000 bp) was divided into sequential non-overlapping 50-bp bins. The number of mutations for each 50-bp bin is plotted. Mutations from two replica crosses for each construct were analysed together. (d) Mutation profiles for repeat constructs ii–vii. Each profile is based on 24 spores (ii, iii, v, vi and vii) or 30 spores (iv) from one representative cross. NA, not applicable. Figure 7: Repeat-induced point mutation (RIP) depends on global disposition of interacting repeats. ( a ) Analysed constructs contain one or more of the following elements positioned, as shown, to either side of a 707-bp or a 303-bp linker region (grey): 337 bp of perfect homology (turquoise) in direct or inverted orientation; 500 bp of partial homology 4H-7N (blue and blue/white) in direct or inverted orientation, either alone or adjacent to 337 bp of perfect homology in inverted orientation, and with or without 22 bp of random sequence inserted between the perfect and partial homology segments. ( b ) The number of mutations within the partial homology repeat (left panel) and the perfect homology repeat (right panel) in the invariant region. For (ii-vii), corresponding mutation profiles shown in d . *** P <0.001; ** P <0.01; NS, P ≥0.05; ns, P -value fluctuates around 0.05. Error bars represent s.e.m. ( c ) Mutation density profiles for constructs (v) and (vii) reveal the effect of the 22-bp insertion at junction between perfect and imperfect inverted repeat units. The invariant region (1,000 bp) was divided into sequential non-overlapping 50-bp bins. The number of mutations for each 50-bp bin is plotted. Mutations from two replica crosses for each construct were analysed together. ( d ) Mutation profiles for repeat constructs ii–vii. Each profile is based on 24 spores (ii, iii, v, vi and vii) or 30 spores (iv) from one representative cross. NA, not applicable. Full size image To further investigate this possibility, we introduced a 22-bp segment of random sequence between perfect and partial homologies, thus interrupting their co-alignment ( Fig. 7a ; constructs v versus vii). In this situation, RIP levels were significantly decreased throughout the region, with the strongest effect observed in the partially homologous segment ‘distal’ to the interruption ( Fig. 7c ). This result reinforced the importance of continuous co-alignment for RIP. However, segments to either side of the insert still exhibited mutation well above background, suggesting the existence either of multiple alignment blocks and/or synergistic but non-simultaneous interactions ( Fig. 7b,d ). Our results corroborate previous findings on somatic chromosome pairing in budding yeast [37] and suggest that an array of direct interactions between co-aligned DNA double helices provides sufficient information for determining their mutual sequence identity ( Fig. 8 ). Our results are consistent with an earlier observation made by Selker and colleagues concerning the lower sensitivity of RIP to sequence divergence between tandem repeat units compared with premeiotic intrachromosomal recombination [38] . Indeed, we have found that repeat segments sharing gross homology of only 25% (3H-9N, Fig. 5b,c ) are efficiently recognized by RIP once their pairing has been induced by the adjacent region of perfect homology. Also consistent with this idea is the fact that we observed no intrachromosomal recombination among many sequenced direct repeats: the majority of them contained 220 bp of perfect homology separated by 0.7 kbp of partial or random homology that should have represented a suboptimal substrate for premeiotic recombination in N. crassa [39] . Our ability to detect mutation of repeats as short as 155 bp, considerably smaller than the previously established threshold of 0.4 kbp (ref. 39 ), is likely due to a combination of several factors, including the high sensitivity of our RIP assay and the nature of repeats units, one of which overlaps a transcription start site of a moderately expressed gene ( NCU00725 ) and therefore could contain fewer stably bound nucleosomes that may need to be remodelled before/during DNA–DNA pairing [40] . 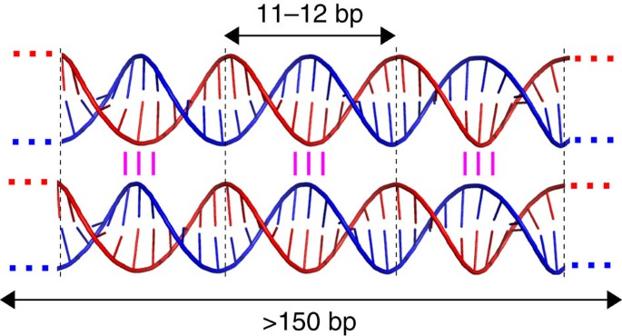Figure 8: A cartoon representing sequence-specific association of double helices of DNA by interactions between periodically spaced trinucleotides. Two intact DNA helices longer than 150 base pairs can engage in stable sequence-specific interactions once every turn and over many turns. Figure 8: A cartoon representing sequence-specific association of double helices of DNA by interactions between periodically spaced trinucleotides. Two intact DNA helices longer than 150 base pairs can engage in stable sequence-specific interactions once every turn and over many turns. Full size image We favour the notion that the elementary unit of homology recognition for RIP is a triplet of DNA base pairs. This possibility brings RIP in line with other nucleic acid matching processes in which triplet interactions have prominent roles, most notably codon/anticodon pairing in the ribosome and DNA/DNA homology recognition catalysed by RecA family proteins. The exact nature of intermolecular interactions remains to be determined. One proposed model, interwrapping of two negatively supercoiled DNA duplexes [18] does not appear likely because it is expected to require homology tracts of at least 5 bp (half a turn of B-DNA), rather than the minimal 3-bp unit defined here. Two other, related, models invoke sequence-specific paranemic pairing as discussed by McGavin [28] and Wilson [29] . Although these models did not specifically address pairing by short periodic units of homology, they emphasized the exclusive property of identical base pairs to form four-strand ‘quartet’ structures, which is attractive because such quartets may provide a robust molecular signature for yet unknown protein factors. We also note that, although all indications point to the intact nature of paired duplexes, involvement of DNA degradation or strand exchange via Watson–Crick base pairing will be rigorously excluded only when the actual mechanism of RIP has been determined. In future, it will be important to understand how homology sensing occurs in the context of chromatin. It remains to be determined whether RIP involves intrinsically nucleosome-free regions, active nucleosome remodelling or post-replicative regions where nucleosomes are not yet restored. The present study has focused only on the basis for homology recognition per se and has excluded only one specific molecule, RAD51, as a potential participant. RID may also be involved in homology sensing in addition to its other roles, and RIP components may also include other, unknown proteins and/or RNA (for example, long non-coding RNAs). In summary, the presented results advance the notion that intact DNA duplexes can pair in vivo , and provide a new perspective from which to further analyse the basis for recombination-independent recognition of homology that underlies not only RIP but also, potentially, other phenomena where pairing of intact homologous chromosomal regions is observed. Media and reagents Cyclosporin A was purchased from Sigma (cat. no. 30024); 50 × Vogel's salts and Ignite were purchased from the FGSC [22] . Synthetic crossing (SC) medium was prepared as described [41] , except that a tenfold higher concentration of biotin was used. Strains The following strains were obtained from the FGSC [22] : 2489 (wild type, mat A ), 4200 (wild type, mat a ), 9720 ( Δku80, his-3, mat A ), 12433 ( Δmei-3::HygR, mat a ), 12434 ( Δmei-3::HygR, mat A ) [23] , 12440 ( Δspo11::HygR, mat A ) and 12441 ( Δspo11::HygR, mat a ). Sequence design of partial homologies 200-bp test segments of partial homology were designed by replacing each designated base in the reference sequence with a randomly chosen alternative base. Each test segment (except 3H-1N-3H-4N) was created de novo in its entirety. 3H-1N-3H-4N was made by substituting the fourth position of every 7-bp homology tract in the test segment 7H-4N. Candidate sequences with inappropriate restriction sites, homonucleotide tracks or GC content deviating from the reference by more than 1% (checked at the level of the entire segment) were excluded. DNA was ordered as ‘gBlocks’ from Integrated DNA Technologies. A[19] was ordered from Integrated DNA Technologies as ‘Ultramer Oligo’. It was designed to contain (dA:dT) 20 , but the cloned fragment appeared to have 19 dA:dT units instead of 20. Sequences of all test segments examined in this study ( Supplementary Data 1 ) as well as complete annotated plasmid maps ( Supplementary Data 2 ) are provided. Transformation by homologous recombination Conidiated recipient strains were kept in 16 × 150-mm glass culture tubes at −20 °C until needed. Each tube provided material for three transformations. 1 M sorbitol was added to each culture tube, and macroconidia were resuspended by vortexing. Suspensions were filtered, split into three 1.7-ml tubes, concentrated by centrifugation into 20 μl, pre-incubated with 1 μg of linearized plasmid DNA on ice for 30 min and electroporated (0.2 mm cuvettes, 1.5 kV, 25 μF, 200 Ω). Ice-cold 1 M sorbitol was added immediately after electroporaion, and macroconidia were plated directly on 3% sorbose agar containing histidine and cyclosporin A. Cyclosporin-resistant colonies were screened by PCR and correct integration events were confirmed by sequencing. Because inactivation of the csr-1 gene was used as a positive selectable marker, only homokaryotic transformants were produced by this procedure [24] . Crosses Crosses were setup at room temperature in 16 × 150-mm glass culture tubes containing 1 × SC medium and 2% sucrose solidified with 2% agar. Except when noted otherwise, the wild-type mat a strain FGSC #4200 was used as a female parent by pre-growing it on SC agar for 4 days to induce formation of protoperithecia. Once aerial hyphae were removed with a cotton tip, macroconidia produced by an appropriate primary transformant were added as a freshly made suspension in distilled water. Developing perithecia were observed on the second day after fertilization, and spores typically started to discharge on the 8th day after fertilization, accumulating on the opposite side of the glass culture tube. For quantitative mutation analysis, spores released by the 13th day after fertilization were removed, and crosses were allowed to mature for another 10 days, after which ‘late’ spores were collected into distilled water. Each culture tube contained 100–200 mature perithecia if biotin was added in tenfold excess, thus corresponding to more than 10 3 independent RIP lineages per cross [42] , [43] , [44] . Two to three independent crosses were analysed for each critical repeat construct as detailed in Table 1 and exemplified in Supplementary Fig. 3 . Spore germination and sampling The fixed sample size of 24 spores per cross could adequately capture variation in mutation counts. In situations where the expected mutation count was low, the fixed sample size of 30 spores per cross was used. Several thousand ascospores were taken from each cross culture tube and heat-shocked for 30 min at 60 °C. Spore suspensions were mixed vigorously, diluted and plated directly on 3% agar, containing 2% sorbose, 0.1% dextrose, 0.5 mg ml −1 histidine and 5 μg ml −1 cyclosporin A. Plates were incubated at 30 °C for 1.5 days, randomly chosen colonies were bored out with sterile glass Pasteur pipettes and transferred into 16 × 150-mm glass culture tubes containing 2 ml of 1 × Vogel medium supplemented with sucrose and histidine. The investigator (E.G.) was not blinded. DNA extraction After growing for 36–40 h on a rolling wheel, mycelial mats were transferred into 1.5-ml microcentrifuge tubes, submerged in liquid nitrogen for a few seconds and crushed with a sterile blue polypropylene pestle (Sigma, cat. Z359947) by gently and repeatedly hitting it with a microcentrifuge tube rack, and digested for 2–3 h in 0.4 ml of solution (100 mM NaCl, 50 mM Tris-HCl pH 8.0, 10 mM EDTA, 1% SDS, 1 mg ml −1 Proteinase K). Digestion reactions were centrifuged for 5 min at 20,000 g to pellet debris, clear supernatant was transferred into a fresh microcentrifuge tube with a wide-bore pipette tip, extracted with phenol-chloroform once, precipitated with 0.3 ml of isopropanol, washed with 75% ethanol once, air-dried, resuspended in 70–100 μl of 10 mM Tris-HCl pH 7.5, and stored at −80 °C. 1:10 dilutions of DNA extractions in water were used for PCR. PCR and sequencing All primer sequences are given as 5′→3′. Constructs with direct repeats were PCR-amplified with the following primer pairs: TCGCCATAAACTCCTCCAGAAT/TGCCCTGTCTATGATATGTGC (155–802 bp perfect repeats), and GCTACCGCCATACGAAGTGTT/TGCCCTGTCTATGATATGTGC (200+220 bp bipartite repeats). Because inverted repeats could not be amplified as a single continuous fragment, external primers were used in combination with primers annealing in the linker region to yield two separate partially overlapping PCR products: PCR product #1: primers GCTACCGCCATACGAAGTGTT and AACGATGGAAATCTGCTACACG; PCR product #2: primers CGCTTCCATGCATTTTGGATG and TGCCCTGTCTATGATATGTGC. Purified PCR products were sequenced directly with Taq DiDeoxy Terminator cycle chemistry and run on 3730XL DNA Analyzer (Applied Biosystems) at the DNA Core Facility (Massachusetts General Hospital, Boston, MA). Sequence and statistical analysis Individual contigs were assembled using phred/Phrap and inspected manually in consed. No assembled contigs were excluded from the analysis. All sequenced contigs are provided ( Supplementary Data 3 ). Contigs were aligned to the parental sequence using clustalw. All sequence alterations, including RIP mutations, were recorded and analysed by a series of custom-built Perl scripts. RIP mutations were counted over regions of interest, and empirical distributions of mutation counts were compared by the K-S test. A custom Python script was used to calculate the K-S statistics and the associated exact P -value by permutation with 10 5 trials ( Supplementary Data 4 ). The average number of mutations per spore was expressed as the mean and as the median. Standard error of the mean (s.e.m.) was computed for the mean number of mutations per spore. S.e.m. values indicate that the variances were similar among compared groups. Pearson’s correlation analysis and Fisher’s Exact test were done in R. Constructing Δspo11 Δmei-3 strains Germinated spores from a cross between strains FGSC #12440 and FGSC #12433 were genotyped at MatA-1 , Mei-3 and Spo11 loci. One Δspo11, Δmei-3, mat a strain (SR0) and one Δspo11, Δmei-3, mat A strains (SR1) were chosen for further analysis. Constructing a repeat cassette for ectopic transformation Plasmid pEAG40 was created by inserting two sequence tags, site A (5′-ACCTCAACCTCAACCCTATCCAC-3′, between Kpn I and Hin cII) and site B (5′-TTCTCTACTTACCACACTACTCATC-3′, between Xba I and Sac I) into pBlueScriptII. A 800-bp fragment of AvHsp82-1 (ref. 36 ) was amplified with primers 5′-CGATCAGGTACACGTGCATT-3′ and 5′-AATAAT GAATTC GGCATTAATTCTTCGCAGTTTTCC-3′ from genomic DNA of Adineta vaga (Metazoa, Bdelloidea) and inserted into pEAG40 between Hin cII and Eco RI to create pEAG44. A 1-kbp fragment of AvHsp82-1 containing the previously cloned 800-bp fragment was amplified with primers 5′-AATAAT GAATTC TACTGATCCAACTAAACTTGATA-3′ and 5′-AATAAT TCTAGA GGCATTAATTCTTCGCAGTTTTC-3′ and inserted into pEAG44 between Eco RI and Xba I cites to create pEAG45. A fragment of pBARKS1 (refs 45 , 46 ) was amplified with primers 5′-ATTATT GAGCTC GACAGAAGATGATATTGAAGG-3′ and 5′-ATTATT GAGCTC TCAGATCTCGGTGACGGGC-3′ and inserted into pEAG45 digested with Sac I to create pEAG50. Genotyping The following primer pairs were used: Spo11 /NCU01120 (5′-GTGTCGGAAGTCCCATTACCA and 5′-GTGACGCTGTGTAGTCGCTTG-3′), Mei-3 /NCU02741 (5′-ACGACAGCGGGATACCAAAC and 5′-TTCGGGCTAGGATCACCAAT-3′), MatA-1 /NCU01958 (5′-GAAGAAGGTCAACGGCTTCA-3′ and 5′-AGAGCCATGTTGTAAGGGTCA-3′), RID /NCU02034 (5′-CCCATTTCCCTCACCAACTCAT-3′ and 5′-GTGGGTGGAAATGCGGTTATTG-3′) and Dp::BAR (5′-GGCGATTAAGTTGGGTAACGC-3′ and 5′-TCACCGCCTGGACGACTAAAC-3′). Assaying histidine sensitivity of Δmei-3 strains Histidine sensitivity [47] of parental mei-3 strains was assayed by inoculating 3 μl of macroconidial suspension in the centre of a 100-mm Petri dish containing 1 × Vogel’s medium with or without 0.5 mg ml −1 histidine. All dishes were placed at 37 °C, once the mycelial front advanced for more than 10 mm from the centre, its location was recorded on the bottom of the dish, and then again 7 h later, from which growth rates were calculated by measuring the radial distance at six randomly chosen directions. Histidine sensitivity of mei-3 cross progeny was assayed by plating heat-shocked spores en masse on 1 × Vogel’s agar with or without histidine and observing germination and growth at 37 °C. Assaying the role of MEI3 in RIP pEAG50 was linearized with ScaI and electroporated into macroconidia of SR0 ( Δspo11, Δmei-3, mat a ). Ignite-resistant transformants [45] were genotyped for the presence of a stably integrated full-length repeat cassette, and one transformant (SR0/T232.2) was chosen for further analysis. SR0/T232.2, pre-grown on 1 × SC medium for 4 days, was fertilized by macroconidia of strains FGSC #2489, FGSC #12440 or SR1. Sixteen-day-old perithecia were crushed in a 1.7-ml centrifuge tube under 100 μl of distilled water, spores were induced by heat and plated, together with broken heat-inactivated perithecial tissues, directly on 3% sorbose agar. All germinated spores were genotyped at Spo11 , Mei-3 and Dp::BAR loci. PCR-amplified Dp::BAR DNA was purified, sequenced directly by primer walking, assembled manually and analysed for the presence of mutations as described. How to cite this article: Gladyshev, E. and Kleckner, N. Direct recognition of homology between double helices of DNA in Neurospora crassa. Nat. Commun. 5:3509 doi: 10.1038/ncomms4509 (2014).